Experimental demonstration of delayed-choice decoherence suppression Wheeler’s delayed-choice experiment illustrates vividly that the observer plays a central role in quantum physics by demonstrating that complementarity or wave–particle duality can be enforced even after the photon has already entered the interferometer. The delayed-choice quantum eraser experiment further demonstrates that complementarity can be enforced even after detection of a quantum system, elucidating the foundational nature of complementarity in quantum physics. However, the applicability of the delayed-choice method for practical quantum information protocols continues to be an open question. Here, we introduce and experimentally demonstrate the delayed-choice decoherence suppression protocol, in which the decision to suppress decoherence on an entangled two-qubit state is delayed until after the decoherence and even after the detection of a qubit. Our result suggests a new way to tackle Markovian decoherence in a delayed manner, applicable for practical entanglement distribution over a dissipative channel. Complementarity normally refers to the wave–particle dual nature in quantum physics. In the delayed-choice experiment proposed by Wheeler, the choice to observe the wave or particle nature is delayed until after the quantum system has already entered the interferometer [1] , [2] . It is even possible to delay the choice after detection of the quantum system by using an ancilla entangled with the quantum system [3] , [4] , [5] , [6] . For example, a delayed-choice quantum eraser is proposed and demonstrated, where the decision of whether to read out or erase the which-path information can be delayed till after the registration of the quanta [3] , [4] . Recently, experiments to investigate the intermediate behaviour between wave and particle nature have been proposed and demonstrated [5] , [6] , [7] . It is also recently shown that entanglement swapping, quantum walk and uncertainty principle can be demonstrated using delayed-choice method [8] , [9] , [10] , [11] , [12] . Although the fundamental aspects of delayed-choice experiments have been well studied, practicality of the delayed-choice method was rather obscure. An intriguing question may arise as to whether the concept of delayed-choice can be adopted for quantum information protocols such as suppressing decoherence, which is a central problem in emerging quantum technology [13] , [14] , [15] . This is a particularly interesting question for Markovian decoherence. Markovian decoherence is considered to be difficult to tackle once the decoherence takes place, since a posteriori methods such as rephasing [16] , [17] or dynamical decoupling [18] , [19] cannot be used. In this Article, we propose and experimentally demonstrate a delayed-choice decoherence suppression scheme by using photonic polarization qubits. In contrast to the normal decoherence suppression scheme [20] , [21] , [22] , [23] , in which the choice whether or not to suppress decoherence is naturally made before the decoherence by the initial weak measurement (WM), our decoherence suppression scheme delays the choice after the decoherence itself. We demonstrate that although the choice to suppress decoherence is made by delayed WM after the decoherence and even after detection of the quantum system, our scheme can suppress decoherence successfully. Schematic and theory The delayed-choice decoherence suppression scenario is schematically shown in Fig. 1a . A two-qubit entangled state, , is prepared at the time t =0 and sent to Alice and Bob with temporal delays and , respectively. At time t D , Bob’s qubit suffers from Markovian amplitude damping decoherence [15] , which is described by a quantum map: , where D is the magnitude of amplitude damping, and subscript S (E) refers to system (environment). 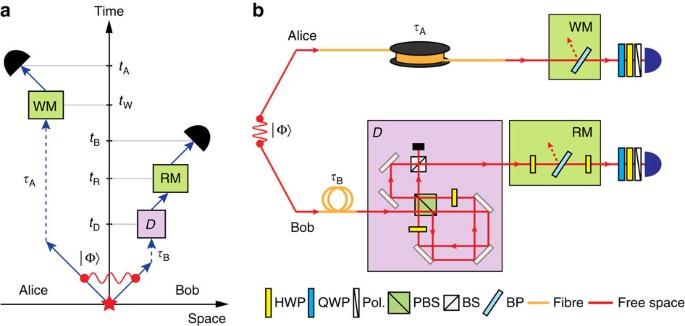Figure 1: Scheme for delayed-choice decoherence suppression. (a) A two-qubit entangled state is prepared and sent to Alice and Bob. In Bob’s quantum channel, amplitude damping decoherence of strengthDis present at timetD, causing reduction of entanglement between the two qubits. Bob performs the RM on his qubit after the decoherence. Alice’s decision whether to suppress the decoherence, by applying the WM on her qubit, may be made after the decoherence or even after the detection of Bob’s qubit. (b) Experimental schematic of delayed-choice decoherence suppression. BP, Brewster’s angle glass plate; BS, non-polarizing beam splitter; HWP, half-wave plate; PBS, polarizing beam splitter; Pol, polarizer; QWP, quarter-wave plate. As a result, the two-qubit state becomes mixed, causing reduced entanglement quantified by concurrence, C d Figure 1: Scheme for delayed-choice decoherence suppression. ( a ) A two-qubit entangled state is prepared and sent to Alice and Bob. In Bob’s quantum channel, amplitude damping decoherence of strength D is present at time t D , causing reduction of entanglement between the two qubits. Bob performs the RM on his qubit after the decoherence. Alice’s decision whether to suppress the decoherence, by applying the WM on her qubit, may be made after the decoherence or even after the detection of Bob’s qubit. ( b ) Experimental schematic of delayed-choice decoherence suppression. BP, Brewster’s angle glass plate; BS, non-polarizing beam splitter; HWP, half-wave plate; PBS, polarizing beam splitter; Pol, polarizer; QWP, quarter-wave plate. Full size image Bob’s reversing measurement (RM), applied immediately after the decoherence, is represented as , where and p r is strength of the RM. Alice’s decision at time t W whether to suppress the decoherence, by applying the WM on her qubit, may be made after the decoherence ( t W > t D ) or even after the detection of Bob’s qubit ( t W > t B ). Alice’s WM is represented as , where and p is WM strength. The reversing measurement strength is chosen to be p r = p + D (1− p ) (refs 20 , 21 , 23 ). After Alice’s WM and Bob’s RM, entanglement in the two-qubit is quantified by concurrence C r (H.-T.L., J.-C.L., K.-H.H. and Y.-H.K., manuscript in preparation), Note that C r > C d that indicates that the delayed-choice decoherence suppression scheme can successfully circumvent Markovian amplitude damping decoherence. It is worth pointing out that, since the WM and RM are both non-unitary, the success probability of our scheme is less than unity. The success probability of the delayed-choice decoherence suppression scheme is (refs 21 , 23 ). Experimental implementation The experimental schematic of delayed-choice decoherence suppression is shown in Fig. 1b . The qubit is encoded in a polarization state of a single-photon: |0›≡| H ›, |1›≡| V ›, where | H › is horizontal polarization and | V › is vertical polarization. The initial two-qubit entangled state (|Φ› with ) is prepared by using type-I spontaneous parametric down conversion from a 6-mm thick β -BaB 2 O 4 crystal [24] . The photons are frequency filtered by a set of interference filters with 5 nm bandwidth. Optical delays and are implemented with single-mode fibres (SMF). Note that wave plates are used to compensate polarization rotation by SMFs at each SMF output. The Markovian amplitude damping decoherence ( D ) is set up with a displaced Sagnac interferometer [21] , [23] . The WM and the RM are implemented with wave plates and Brewster’s angle glass plates [25] . The final two-qubit state is analysed with wave plates and polarizers via two-qubit quantum state tomography [23] . We implement the delayed-choice decoherence suppression scheme in two configurations, space-like separation and time-like separation, by varying the temporal delays and . The space–time diagrams for the two configurations are shown in Fig. 2 . First, in Fig. 2a , we set up the temporal delays such that Alice’s WM and Bob’s decoherence events are in space-like separation. To make sure that the delayed-choice is indeed made after the decoherence itself, we need to consider the timing resolution of the detector (0.35 ns), the coincidence time window for measuring the joint detection events (2.0 ns) and the physical dimensions of the apparatus implementing WM, RM and D . The times for the photon to traverse the apparatus implementing WM, RM and D are 0.10, 0.33 and 1.0 ns, respectively. The overall timing uncertainty is thus 3.8 ns. Since Alice’s WM is made 5.3 ns after the decoherence event, it can be guaranteed that no information about Alice’s choice can be transferred to Bob at the time of decoherence. Furthermore, Alice’s WM and Bob’s decoherence are physically separated by L =2.8 m, so that the time difference between the two events is shorter than the time at which light travels between them (5.3 ns< L/c =9.3 ns). The two events are, thus, in space-like separation as neither of the events are within the forward light cones of each other, see Fig. 2a . This ensures that no causal relationship, that is, no classical communication, can be established between the two events in this setting. 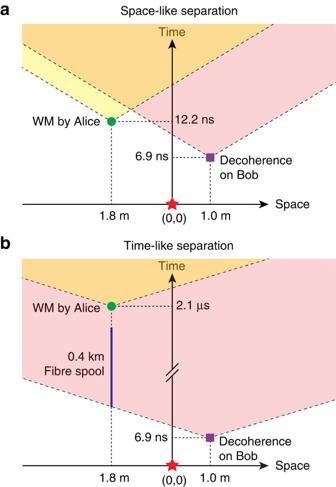Figure 2: Space–time diagrams for space-like and time-like configurations. The two-qubit entangled state generation event is marked as a red star at the origin. The spatial separation between the two events, that is, the decoherence on Bob’s qubit and WM on Alice's qubit, isL=2.8 m. The shaded regions represent forward light cones of the events. (a) The two events are space-like separated. The temporal difference between the two events (5.3 ns) is shorter than the time light travels between them (L/c=9.3 ns). The two events are thus not in a causal relation, that is, no classical communication is possible between the two events. (b) The two events are time-like separated: WM on Alice’s qubit is in the time-like future of the decoherence event on Bob’s qubit. Figure 2: Space–time diagrams for space-like and time-like configurations. The two-qubit entangled state generation event is marked as a red star at the origin. The spatial separation between the two events, that is, the decoherence on Bob’s qubit and WM on Alice's qubit, is L =2.8 m. The shaded regions represent forward light cones of the events. ( a ) The two events are space-like separated. The temporal difference between the two events (5.3 ns) is shorter than the time light travels between them ( L/c =9.3 ns). The two events are thus not in a causal relation, that is, no classical communication is possible between the two events. ( b ) The two events are time-like separated: WM on Alice’s qubit is in the time-like future of the decoherence event on Bob’s qubit. Full size image Second, we set up the apparatus such that Alice’s WM is in time-like future of the decoherence event on Bob, see Fig. 2b . Experimentally, we increase by inserting a 400-m fibre spool on Alice’s side to achieve . As with the space-like separation depicted in Fig. 2a , Alice’s WM is made sufficiently after the decoherence itself, hence no information about Alice’s choice can be sent back to Bob’s decoherence event. In the time-like separation, however, it is possible for Bob to send classical information about the decoherence to Alice, possibly affecting Alice’s WM. The delayed-choice decoherence suppression is demonstrated in Fig. 3 . We first fixed the magnitude of decoherence to be D =0.617 and varied the WM strength p and monitored the concurrence of the final two-qubit state, see Fig. 3a . The concurrence increases as the WM strength increases. For both space-like separation shown in Fig. 2a and time-like separation shown in Fig. 2b , the decoherence is successfully circumvented by using our delayed-choice decoherence suppression scheme. Then we set the WM strength at P =0.617 and observe the concurrence as D increases, see Fig. 3b . When the two-qubit system is subject to decoherence, entanglement of the system significantly degrades as D becomes large. However, when the delayed-choice decoherence suppression scheme is applied, more entanglement is shared by Alice and Bob, as evidenced in higher concurrences ( C r > C d ). This again confirms that it is indeed possible to perform delayed-choice decoherence suppression. 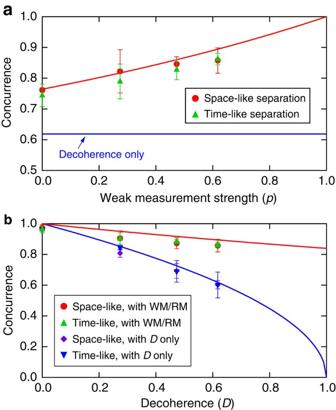Figure 3: Experimental concurrence for the space-like and time-like separation experiments. (a) As a function of WM strength forD=0.617. (b) As a function of decoherence with or without WM/RM (P=0.617). The results show that our delayed-choice decoherence suppression scheme is able to recover entanglement. Note that both space-like and time-like separation experiments give the same results. The solid lines represent the theoretical curves forCdandCr. The error bars represent the statistical error of ±1s.d. Figure 3: Experimental concurrence for the space-like and time-like separation experiments. ( a ) As a function of WM strength for D =0.617. ( b ) As a function of decoherence with or without WM/RM ( P =0.617). The results show that our delayed-choice decoherence suppression scheme is able to recover entanglement. Note that both space-like and time-like separation experiments give the same results. The solid lines represent the theoretical curves for C d and C r . The error bars represent the statistical error of ±1s.d. Full size image Our decoherence suppression scheme can be applicable to practical entanglement distribution scenarios, an example of which is shown in Fig. 4 . First, Alice generates N identical pairs of entangled qubits and shares it with Bob through a quantum channel that has unknown amplitude damping decoherence in the channel, see Fig. 4a . The decoherence causes the two-qubit state to become a mixed state ρ d and lowers concurrence. Alice and Bob store the qubits in quantum memories to use it on demand. Alice and Bob do not know the existence of decoherence in advance and the ensemble of quantum states shared by Alice and Bob is , see Fig. 4b . Bob then uses a small subset of his qubits to estimate the magnitude of decoherence D by monitoring the weight between |0›‹0| and |1›‹1|. Assuming the initial state |Φ› with , the quantum state of Bob’s qubit after decoherence is . As Bob makes m independent measurements, the variance of Bob’s estimation of D is . Bob then uses a classical communication channel to inform the measured D value to Alice. Now, Alice and Bob share N − m identical pairs of partially entangled qubits with known D , see Fig. 4c . The delayed-choice decoherence suppression scheme can be applied with a reversing measurement strength ρ r (refs 20 , 21 , 23 ). As a result, the two parties now share highly entangled qubits, with concurrence C r , while the final number of qubits is decreased to ( N − m ) P S due to Bob’s estimation of D and success probability P S of the scheme. Our delayed-choice decoherence suppression scheme provides a new strategy for entanglement distillation over a decoherence channel. 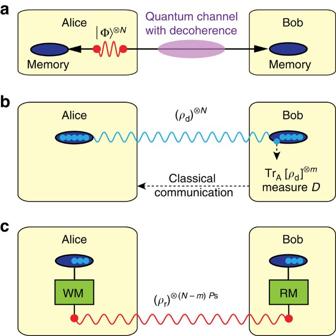Figure 4: Entanglement distribution using delayed-choice decoherence suppression. (a) Alice sharesNidentical pairs of entangled qubits |Φ› with Bob by a quantum channel which has amplitude damping decoherence with unknownD. Alice and Bob store their own qubits in their quantum memories for later use. (b) Bob usesmqubits to measure the magnitude of decoherenceDand inform the value ofDto Alice via classical communication. (c) Alice and Bob apply delayed-choice decoherence suppression scheme: Alice executes delayed WM to her qubit, while Bob makes RM to his qubit. As a result, Alice and Bob share highly entangled qubits. Figure 4: Entanglement distribution using delayed-choice decoherence suppression. ( a ) Alice shares N identical pairs of entangled qubits |Φ› with Bob by a quantum channel which has amplitude damping decoherence with unknown D . Alice and Bob store their own qubits in their quantum memories for later use. ( b ) Bob uses m qubits to measure the magnitude of decoherence D and inform the value of D to Alice via classical communication. ( c ) Alice and Bob apply delayed-choice decoherence suppression scheme: Alice executes delayed WM to her qubit, while Bob makes RM to his qubit. As a result, Alice and Bob share highly entangled qubits. Full size image In summary, we have proposed and experimentally demonstrated the delayed-choice decoherence suppression in which the choice whether to suppress decoherence is made after the decoherence and even after the detection of a qubit. It is interesting to note that our delayed-choice decoherence suppression scheme allows to circumvent Markovian amplitude damping decoherence, even though the decision to suppress the decoherence made after the decoherence itself. While the demonstration in this paper utilized photonic polarization entanglement, the delayed-choice scheme demonstrated in this work can be generalized and applied to other quantum systems. Our result thus provides a new direction in tackling decoherence in a delayed manner and has important implications in practical implementations of various quantum information protocols. How to cite this article: Lee, J.-C. et al. Experimental demonstration of delayed-choice decoherence suppression. Nat. Commun. 5:4522 doi: 10.1038/ncomms5522 (2014).